Rapid fabrication of hierarchically structured supramolecular nanocomposite thin films in one minute Functional nanocomposites containing nanoparticles of different chemical compositions may exhibit new properties to meet demands for advanced technology. It is imperative to simultaneously achieve hierarchical structural control and to develop rapid, scalable fabrication to minimize degradation of nanoparticle properties and for compatibility with nanomanufacturing. Here we show that the assembly kinetics of supramolecular nanocomposites in thin films are governed by the energetic cost arising from defects, the chain mobility and the activation energy for inter-domain diffusion. By optimizing only one parameter, the solvent fraction in the film, the assembly kinetics can be precisely tailored to produce hierarchically structured thin films of supramolecular nanocomposites in one minute. Moreover, the strong wavelength-dependent optical anisotropy in the nanocomposite highlights their potential applications for light manipulation and information transmission. The present study may open a new avenue in designing manufacture-friendly continuous processing for the fabrication of functional nanocomposite thin films. Developments in colloidal particle synthesis enable one to engineer nanoparticles with controlled size, shape and chemical composition [1] , [2] , [3] , [4] , [5] , [6] , [7] . Numerous studies have demonstrated the significant impact of nanoparticle-based materials in life sciences, microelectronics, light manipulation, energy harvesting and storage [8] , [9] , [10] . Co-assemblies of nanoparticles and organic building blocks clearly hold promise for generating nanocomposites using different elements on the periodic table that combine the advantages of both families of building blocks [11] , [12] , [13] , [14] , [15] . To fulfill these promises, at least two requirements must be satisfied. One is to control the spatial arrangement of nanoparticles spanning multiple length scales in a reproducible manner, so as to modulate inter-particle coupling and the collective properties of nanocomposites [16] , [17] , [18] , [19] , [20] , [21] . The other is to understand and manipulate the kinetics of the assembly process to ensure compatibility with existing fabrication infrastructures. To be relevant, the fabrication process must be rapid, completed within a few minutes to minimize degradation of nanoparticle properties because of exposure to the processing environment and for compatibility with nanomanufacturing [22] . In comparison to many current approaches such as DNA and controlled solvent evaporation, block copolymers (BCPs) provide scalable platforms to obtain nanoscopic organization of nanoparticles, but require favourable nanoparticle–polymer interactions to achieve nanoparticle dispersion, and it remains difficult to control inter-particle ordering within BCP microdomains [14] , [23] , [24] , [25] . In addition, their self-assembly processes typically require tens of minutes or hours to complete and can lead to degradation of inherent optoelectronic properties of the nanoparticles. Thermal annealing alone or in conjunction with solvent annealing has been used to accelerate the assembly process, but is not suitable for temperature-sensitive nanoparticles [26] , [27] . BCP-based supramolecules are constructed by non-covalently attaching small molecules to polymer side chains. The presence of small molecules eliminates the need to modify either the nanoparticle ligand or polymer for nanoparticle incorporation and improve inter-particle ordering within BCP microdomains. One-, two- and three-dimensional (3D) nanoparticle arrays can be obtained in thin films of supramolecular nanocomposites via solvent annealing for a range of nanoparticles or nanoparticle mixtures [17] , [19] , [20] , [28] , [29] . Kinetically, the presence of small molecules also provides unique opportunities to manipulate the energy landscape of the assembly process and to accelerate the assembly kinetics so that inherent properties of nanoparticles can be maintained and continuous thin film processing techniques can be implemented for device fabrication. However, the supramolecular nanocomposite has at least five components during solvent annealing, making it extremely challenging to manipulate the assembly process. Here, we systematically analyse the thermodynamics and kinetics of self-assembly in thin films of supramolecular nanocomposite upon exposure to solvent vapour. The assembly kinetics depends on the energetic penalty of the excess interfacial area because of defects, the chain mobility and the activation energy for inter-domain diffusion. It is the solvent content in the film, f s , during solvent annealing, rather than the swelling rate, which governs the ordering kinetics and pathway. By optimizing only one parameter, that is, f s , a marked acceleration in the assembly process can be achieved to generate hierarchically structured nanocomposite films in 1 min. The timescale of ordering process demonstrated here, that is, 1 min, is clearly compatible with many scalable manufacturing processes, such as draw coating, ink-jet printing and roll-to-roll fabrication of functional thin films. Furthermore, upon formation of 3D ordered arrays of gold nanoparticles, nanocomposite thin films exhibit a wavelength-dependent optical anisotropy and a rapid switch of polarization states in the visible light regime, confirming the feasibility to generate new functional materials by forming hierarchically structured nanocomposites. Fabrication of supramolecular nanocomposite thin films The supramolecular nanocomposite is a blend of ∼ 5 nm Au nanoparticles capped with 1-dodecanethiol ( Supplementary Fig. 1 ) and the supramolecule, polystyrene- b -poly-4-vinylpyridine (PS(19 kDa)- b -P4VP(5.6 kDa))(PDP) 1.7 , prepared by hydrogen-bonding 3-pentadecylphenol (PDP) to the 4VP units of a BCP, PS- b -P4VP at a PDP/4VP ratio of 1.7 (ref. 30 ). In thin film, after solvent annealing using chloroform, it forms hexagonally packed 3D nanoparticle arrays where the Au nanoparticles are selectively located at the interstitial sites in the P4VP(PDP) matrix ( Fig. 1 ) [29] . 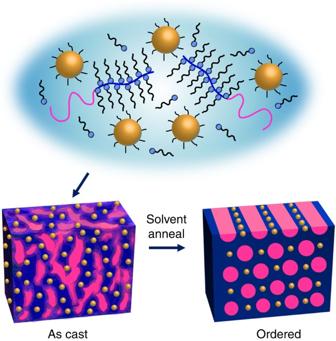Figure 1: Supramolecular nanocomposite thin films. After solvent annealing, the nanocomposite thin film assumes 3D nanoparticle arrays packed in a distorted hexagonal lattice parallel to the surface. Figure 1: Supramolecular nanocomposite thin films. After solvent annealing, the nanocomposite thin film assumes 3D nanoparticle arrays packed in a distorted hexagonal lattice parallel to the surface. Full size image Assembly kinetics during solvent annealing The solvent fraction during solvent annealing, f s , is determined by monitoring film thickness in situ ( Fig. 2a ). 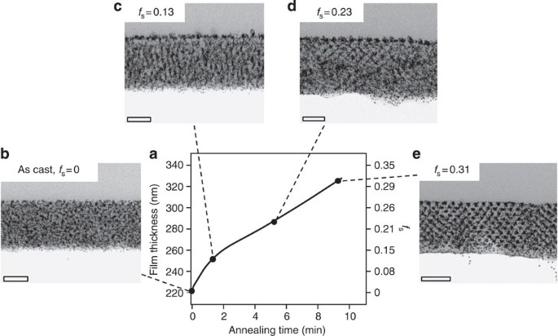Figure 2: Structural evolvement as a function offs. Cross-sectional TEM images of a∼220-nm thin film of a blend of PS(19 kDa)-b-P4VP(5.6 kDa)(PDP)1.7and 6 vol% of∼5 nm Au nanoparticles that was solvent annealed under chloroform vapour at differentfs. The film thickness profile during solvent annealing is shown ina. The film was characterized atfs=(b) 0, (c) 0.13, (d) 0.23 and (e) 0.31, respectively. Scale bar=100 nm. Figure 2b–e shows the cross-sectional transmission electron microscopy (TEM) images of the films quenched at f s =0, 0.13, 0.23 and 0.31, respectively. The diffusion coefficient of CHCl 3 in polymer is ∼ 10 −12 m 2 s −1 (refs 31 , 32 ). The solvent molecules are distributed uniformly in the film for the timescale considered here. The as-spun film is microphase-separated with a poorly ordered structure ( Fig. 2b ). The excess interface resulting from defects results in a sufficient thermodynamic driving force to form ordered nanostructure, provided the components are mobile. Initially, a nanostructure normal to the film surface developed at f s =0.13 ( Fig. 2c ). This can be attributed to the solvent gradient field normal to the surface during spin casting. Upon further annealing at f s =0.23, the supramolecule locally arranged itself and formed distorted hexagonally packed cylinders oriented parallel to the surface and the nanoparticles ordered within the P4VP(PDP) matrix ( Fig. 2d ) [33] . With time, the grain size of the in-plane hexagonal lattice increased from the film surface, resulting in highly ordered hexagonally packed 3D nanoparticle arrays parallel to the surface throughout the film ( Fig. 2e ). Figure 2: Structural evolvement as a function of f s . Cross-sectional TEM images of a ∼ 220-nm thin film of a blend of PS(19 kDa)- b -P4VP(5.6 kDa)(PDP) 1.7 and 6 vol% of ∼ 5 nm Au nanoparticles that was solvent annealed under chloroform vapour at different f s . The film thickness profile during solvent annealing is shown in a . The film was characterized at f s =( b ) 0, ( c ) 0.13, ( d ) 0.23 and ( e ) 0.31, respectively. Scale bar=100 nm. Full size image The ex situ TEM results nicely capture the self-assembly pathway of supramolecular nanocomposites in thin films and can be described in terms of the thermodynamics and kinetics in a qualitative manner. 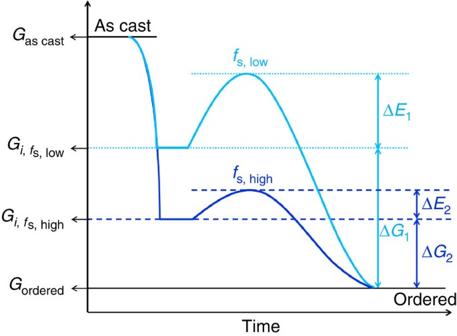Figure 3: Qualitative free energy diagram of the assembly pathway. The as-cast film has the largest value of free energyGas castbecause of the interfacial energy associated with defects. The energy difference between the as-cast and ordered states ΔGis the thermodynamic driving force of the assembly process.Greduces as a function offsas the solvent mediates energy cost of defects. ΔEcorresponds to the activation energy barrier for the supramolecular nanocomposite to order. Figure 3 shows the energy landscape of the assembly process for two solvent fractions f s, low and f s, high . G as cast and G ordered refer to the overall energy of the as-cast film and that of the ordered one. Overall, the main driving force for the structural evolution, that is, the energy difference, Δ G , between the as-cast and ordered films, is to minimize the interfacial area at the defects. Δ G can be approximated as γ. Δ A , where γ is the interfacial energy between PS and P4VP(PDP) 1.7 /nanoparticles and Δ A is the interfacial area because of the defect. , and χ eff =χ o (1— f s ), where χ eff and χ o are the Flory–Huggins interaction parameters of the supramolecule with and without solvent, respectively [34] . As f s, increases, the energetic cost of defects and the thermodynamic driving force to form ordered structure decreases, and thus may lead to a lower assembly rate following the Arrhenius equation. Figure 3: Qualitative free energy diagram of the assembly pathway. The as-cast film has the largest value of free energy G as cast because of the interfacial energy associated with defects. The energy difference between the as-cast and ordered states Δ G is the thermodynamic driving force of the assembly process. G reduces as a function of f s as the solvent mediates energy cost of defects. Δ E corresponds to the activation energy barrier for the supramolecular nanocomposite to order. Full size image Kinetically, the formation of the nanostructure requires the re-arrangement of material in the nanocomposite. The diffusion rate depends on the chain mobility and the energy barrier, Δ E a , for the inter-domain diffusion. The presence of solvent lowers the T g of the supramolecule, which is estimated to be 34.7, 13.4 and 0 °C at f s =0.13, 0.23 and 0.31, respectively [35] . The chain mobility of the supramolecule increases as a function of f s . The diffusion constant of the supramolecular nanocomposite should be similar to that of supramolecule or BCP. At the interface between two blocks, a diffusing chain experiences a uniform potential when diffusing parallel to the interface but a periodic potential for perpendicular diffusion, resulting in an anisotropy in the diffusion coefficients parallel to the interface D para and normal to the interface D perp (refs 36 , 37 , 38 ). D perp follows a hindered diffusion mechanism and is expressed as D perp ∼ exp(−Δ E a ). Δ E a is proportional to χ eff , the enthalpic penalty for pulling one block through the other domain [39] . The anisotropic diffusion explains the assembly pathway observed in the cross-sectional TEM images in Fig. 2 . At low f s , D para is higher than D perp because of the high χ eff and the nanocomposite forms cylinders perpendicular to the surface. As f s increases, χ eff decreases, so the inter-domain diffusion is less costly, allowing the supramolecule and nanoparticles to rearrange and form a parallel cylindrical morphology. 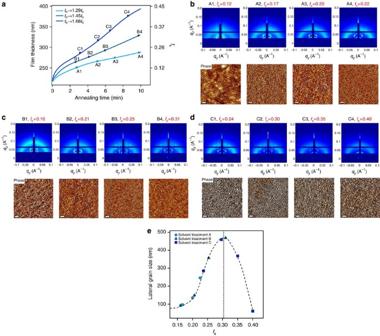Figure 4:In situGISAXS studies on the assembly pathway and kinetics. (a) Film thickness versus time profiles of the∼220 nm nanocomposite thin films annealed under different solvent treatments duringin situGISAXS measurements. Solvent treatments A, B and C allowed the three nanocomposite thin films to reachfs=0.23, 0.31 and 0.40 in 10 min, respectively. The GISAXS patterns and the corresponding AFM phase images during solvent treatments A, B and C at the points indicated inaare shown inb,candd, respectively. (e) The plot of the grain size as a function offs, showing that the ordered nanostructure is optimized atfs=0.31. The dotted line is intended as a visual guide to further elucidate the trend in the grain size change. Scale bar, 100 nm. In situ X-ray scattering measurements Figure 4 shows the in situ grazing incidence small angle X-ray scattering (GISAXS) studies of ∼ 200 nm thin films of PS(19 kDa)- b -P4VP(5.6 kDa)(PDP) 1.7 /5 nm Au nanoparticle blend that underwent three different solvent treatments. The corresponding atomic force microscopy (AFM) images of the films are also shown. The ordering in the as-cast film is poor, as evidenced by the broad Bragg peak and the structure has an overall vertical alignment biased by the solvent field during spin casting. Upon exposure to the solvent under solvent treatment A where f s was increased from 0 to 0.23 in 10 min, the GISAXS pattern A1 at f s =0.12 shows a diffraction ring from the nanostructure ( Fig. 4b ). The corresponding AFM image shows the cylindrical microdomains with different orientations with respect to the interface. When f s is between 0.13 and 0.23, there are two spots of increasing intensity along the first Bragg rod, indicating that the cylindrical microdomains are beginning to align parallel to the surface. At f s =0.23, the scattering pattern corresponds to hexagonally packed nanoparticle arrays oriented parallel to the surface. Under solvent treatment B where f s was increased from 0 to 0.31 in 10 min, the film is allowed to reach a higher f s . In GISAXS pattern B3 at f s =0.25 ( Fig. 4c ), higher order peaks in the diffraction pattern are seen, which shows the completion of the re-orientation of the cylindrical microdomains and the formation of distorted hexagonally packed nanoparticle arrays parallel to the surface. Further annealing ( f s =0.31) leads to a larger grain size of the in-plane morphology evidenced by a set of sharper Bragg diffraction peaks in the GISAXS pattern and the improved long-range order seen in the AFM image corresponding to B4. However, when 0.31< f s <0.35 under solvent treatment C, the GISAXS patterns and the corresponding AFM images indicate that the ordered structure deteriorates and becomes disordered at high f s ( Fig. 4d ). When f s =0.4, the GISAXS pattern at C4 is dominated by the ‘correlation hole’ effect and no clear structure factor features are observed. The lateral grain size for each nanocomposite thin film was estimated using the Scherrer equation and plotted in Fig. 4e as a function of f s . All results fall on one master curve and the largest grain size, ∼ 0.47 μm, is obtained at f s =0.31. Figure 4: In situ GISAXS studies on the assembly pathway and kinetics. ( a ) Film thickness versus time profiles of the ∼ 220 nm nanocomposite thin films annealed under different solvent treatments during in situ GISAXS measurements. Solvent treatments A, B and C allowed the three nanocomposite thin films to reach f s =0.23, 0.31 and 0.40 in 10 min, respectively. The GISAXS patterns and the corresponding AFM phase images during solvent treatments A, B and C at the points indicated in a are shown in b , c and d , respectively. ( e ) The plot of the grain size as a function of f s , showing that the ordered nanostructure is optimized at f s =0.31. The dotted line is intended as a visual guide to further elucidate the trend in the grain size change. Scale bar, 100 nm. Full size image Hierarchically structured nanocomposites in 1 min In addition to f s , the swelling rate is another parameter during the solvent treatments. A series of in situ GISAXS studies were conducted to reach a specific f s at different swelling rates and the grain size was plotted against annealing time for each f s ( Fig. 5a ). The results show a time- f s superposition phenomenon. The system needs longer annealing time to reach an ordered state at relatively low f s as the assembly rate is facilitated by Δ G but limited by Δ E a and chain mobility. Near the optimal f s , the grain growth rate is very fast initially due to the dominant driving force but eventually experiences retardation as a result of the competition between the kinetic terms and Δ G . The results indicate that f s determines the assembly rate and the solvent entry rate has a minimal role in the assembly kinetics. Similar grain sizes of the optimized nanostructure were observed in the film that reached the same f s at three different swelling rates during annealing ( Fig. 5b ). Ordered films of hierarchically structured supramolecular nanocomposite can be readily obtained in 1 min. However, the decreasing Δ G at high f s limits the growth of the nanostructure over micrometer scales. To optimize nanostructure in a short period of annealing time at high f s , the solvent treatment is applied to the nanocomposite film on lithographically patterned surface ( Fig. 5c ). The film reached the optimal f s in 1.5 min during solvent annealing, yielding unidirectional nanoparticle arrays in the nanocomposite film over macroscopic distances in the trenches. 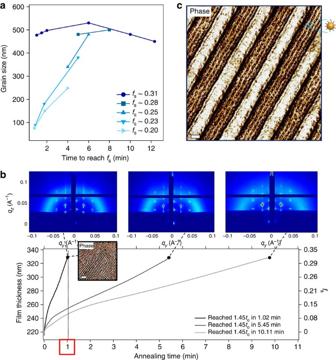Figure 5: Time-fssuperposition during solvent annealing. A series ofin situGISAXS studies were conducted on six identical nanocomposite thin films. (a) The grain size of the nanostructure was plotted against the required annealing time to reach certainfs. (b) The GISAXS patterns of three identical thin films treated with different swelling rates. Hierarchically structured nanoparticle assemblies can be readily obtained in 1 min. (c) AFM phase image of a∼50-nm nanocomposite thin film in lithographically patterned trenches that forms unidirectional nanoparticle arrays over macroscopic distances in 1.5 min. The bright circular dots in the image represent the 5 nm nanoparticles as illustrated by the schematics. Scale bar=100 nm. Figure 5: Time- f s superposition during solvent annealing. A series of in situ GISAXS studies were conducted on six identical nanocomposite thin films. ( a ) The grain size of the nanostructure was plotted against the required annealing time to reach certain f s . ( b ) The GISAXS patterns of three identical thin films treated with different swelling rates. Hierarchically structured nanoparticle assemblies can be readily obtained in 1 min. ( c ) AFM phase image of a ∼ 50-nm nanocomposite thin film in lithographically patterned trenches that forms unidirectional nanoparticle arrays over macroscopic distances in 1.5 min. The bright circular dots in the image represent the 5 nm nanoparticles as illustrated by the schematics. Scale bar=100 nm. Full size image Wavelength dependence optical anisotropy Once the nanocomposite is ordered, the inter-particle distance and coupling are defined, leading to new properties unique to ordered arrays of nanoparticles ( Fig. 6 ) [40] , [41] , [42] , [43] . For the solvent annealed nanocomposite thin films, the in-plane inter-particle distance is 9.6 nm, smaller than that of out-of-plane (26 nm), thereby leading to a stronger in-plane inter-particle plasmonic coupling to the first approximation. Indeed, a wavelength-dependent optical anisotropy was observed and the optical birefringence, Δ n , is close to −0.05 between 400 and 600 nm ( Fig. 6b ). In contrast, the as-cast film mainly consists of randomly distributed Au nanoparticles and is fairly optically isotropic ( Supplementary Figs 2 and 3 ). Different from other materials with optical anisotropy, the refractive indices of the ordered nanocomposite have strong wavelength dependence. The highest Δ n is −0.087 at 544 nm, comparable to that of lithium niobate ( Fig. 6c ). The complex reflectivity ratio ( ρ = r p / r s =tan( Ψ ) e i Δ ) was measured as a function of wavelength to evaluate the optical properties of nanocomposite thin films, where r p and r s are the complex reflection coefficients for p - and s -polarized light and tan(ψ) and Δ are the changes in amplitude and phase between p and s components of polarized light reflected from the film as shown in Fig. 6d,e , respectively. When the incident angle was close to the Brewster angle, θ=55° in this case, the reflection from the film of supramolecule alone is s -polarized over a broad range of wavelength as expected. For nanocomposites, on the contrary, the presence of Au nanoparticles leads to large changes in both tan( ψ ) and Δ ( Fig. 6c ). The wavelength-dependent polarization was clearly seen between 400 and 550 nm for the nanocomposite thin films before and after solvent annealing. Notably, there is a strong blue shift from 457 to 472 nm ( ∼ 15 nm) when Au nanoparticles are rearranged from disordered to ordered arrays. 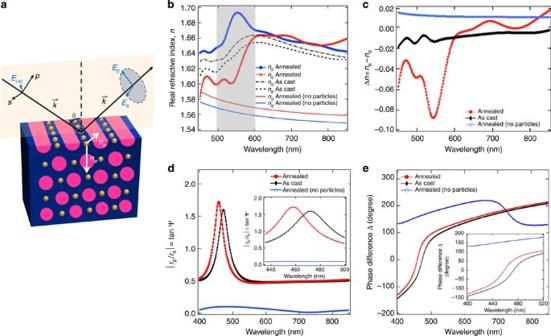Figure 6: Wavelength-dependent optical anisotropy in nanocomposite thin films. (a) Schematics of the ellipsometry measurements of the in-plane (no+iko) and out-of-plane (ne+ike) components of the complex refractive indices. (b) Real refractive index,no, of different films as a function of wavelength. Ordered nanocomposite thin film shows a pronounced peak nearλ=544 nm (highlighted in grey) because of the strong interaction between the incident electromagnetic wave and the collective plasmonic coupling of the ordered nanoparticle chains parallel to the surface. This leads to a wavelength-dependent optical birefringence of the film (Δn∼−0.087 at 544 nm) for light manipulation applications as shown incand a wavelength dependence of the reflectivity ratio and the phase difference shown indande, respectively. Figure 6: Wavelength-dependent optical anisotropy in nanocomposite thin films. ( a ) Schematics of the ellipsometry measurements of the in-plane ( n o + ik o ) and out-of-plane ( n e + ik e ) components of the complex refractive indices. ( b ) Real refractive index, n o , of different films as a function of wavelength. Ordered nanocomposite thin film shows a pronounced peak near λ =544 nm (highlighted in grey) because of the strong interaction between the incident electromagnetic wave and the collective plasmonic coupling of the ordered nanoparticle chains parallel to the surface. This leads to a wavelength-dependent optical birefringence of the film (Δ n ∼ −0.087 at 544 nm) for light manipulation applications as shown in c and a wavelength dependence of the reflectivity ratio and the phase difference shown in d and e , respectively. Full size image Thus, the nanocomposite thin films can polarize lights of different wavelength by simply varying the spatial arrangement of nanoparticles. The Au nanoparticle used here is only 5 nm in size and the edge-to-edge distance between two particles is approximately 3–4 nm. Thus, the plasmonic coupling between the nanoparticles is fairly weak as can be seen in the ultraviolet–visible spectra of the nanocomposite thin films ( Supplementary Fig. 4 ). However, simply by varying the nanoparticle assemblies in thin films via the solvent treatment demonstrated here, the macroscopic optical properties of the nanocomposites can be tailored along different directions. It is worthwhile to note that the dimensions of the nanoparticle arrays are at least one order of magnitude smaller than that of visible wavelength. However, the nanocomposite still exhibits quite large optical anisotropy, clearly demonstrating the potential of supramolecular nanocomposites as metamaterials. More importantly, the spatial arrangement of nanoparticles after annealing leads to anisotropic collective properties with strong wavelength dependence even though the inter-particle coupling is rather weak. Thus, the nanocomposite films presented here open an opportunity to manipulate how light of different wavelength interacts with the film to tune the functional wavelength range of the optical coating. The apparent assembly rate and the pathway in the supramolecular nanocomposite thin film reflect a balance between Δ G , the mobility of the supramolecules and Δ E a , all of which depend on f s . Modulating f s during solvent annealing enables control over the assembly kinetics and pathway in the system. At low f s (for example, f s <0.12), Δ G is large and so is Δ E a . D perp is lower than D para , allowing only short-range diffusion along the interface to improve the perpendicular morphology at intermediate f s (for example, 0.12< f s <0.23), the presence of solvent lowers the Δ E a to make D perp appreciable. As f s approaches an optimal value, in this case f s =0.31, the nanocomposite orders rapidly. At high f s (for example , f s >0.31), Δ G decreases significantly and assemblies with high defect density or in disordered state were observed even though the increased chain diffusion and lowered Δ E a should facilitate the defect annihilation. The processing parameters used for supramolecular nanocomposite thin films may also be applicable to other BCP-based systems. However, to achieve the assembly within the absolute timescale presented here, that is, 1 min, which is required to be compatible with current film processing techniques and on-line continuous fabrication, the following factors are unique to supramolecular systems and need to be taken into consideration to design the nanocomposite. Small molecules were shown to control inter-particle ordering, incorporate functionalities and modulate the local environment of nanoparticles [28] . Here, the presence of PDP modulates the thermodynamics and kinetics and facilitates the fast assembly process during solvent annealing ( Supplementary Fig. 5 and Supplementary Discussion ). PDP molecules form hydrogen bonds with P4VP to change the polymer chain architecture from coil to comb and reduce chain entanglement. Unbound PDP molecules act as a plasticizer to modulate chain mobility and their spatial arrangement influences χ eff . In addition, as PDP has a higher solubility in CHCl 3 than the supramolecule, it can act as a solvent absorber to make the entire film swell faster than those with a lesser amount of or no unbound PDP. Thus, the supramolecular system gains mobility rapidly. In summary, these studies show a comprehensive investigation of the assembly kinetics in the nanocomposite thin films during solvent annealing. By understanding the interplay between the energetic driving forces and kinetic pathways, a fast ordering process with a minimal amount of solvent can be designed to achieve hierarchically structured nanocomposite thin films over macroscopic distances. The mechanism shown provides fundamental guidance for designing manufacturing-friendly processing techniques to enable scalable nanofabrication of nanocomposite-based devices using blade coating, ink-jet printing, and dynamic zone annealing. Furthermore, the wavelength-dependent anisotropic optical properties for 3D ordered arrays of gold nanoparticles clearly demonstrated the potential and feasibility for engineering nanocomposites for light manipulation and require further in-depth investigation. The optical properties of nanocomposite thin films depend on the properties of individual nanoparticles and, equally importantly, well-defined inter-particle distance along different directions. As the supramolecular approach is compatible with nanoparticles of different chemical compositions and can lead to a library of nanoparticle assemblies, present studies clearly open a viable approach to generate a new family of optical coating for light manipulation, wave plates, optical modulators and, potentially, information transmission. Preparation of supramolecular nanocomposite thin films PS(19 kDa)- b -P4VP-(5.2 kDa) (PDI=1.09) was purchased from Polymer Source, Inc. 3-n-Pentadecylphenol (95%) was purchased from Acros. Chloroform was purchased from Fisher. All chemicals were used as received. The Au nanoparticles were synthesized using the method reported by Peng et al . [44] Blends of supramolecules and nanoparticles were prepared as described previously. Thin films were prepared by spin-coating the mixed solutions onto silicon wafers (200 nm thermal oxide/Si) with spinning speeds ranging from 1,000 to 3,000 r.p.m. For solvent annealing, samples were annealed using CHCl 3 injected inside a 250-ml Teflon chamber at room temperature. The amount of solvent injected was varied from 0.3 to 2 ml to tailor the swelling rate. The thickness of the film was monitored using Filmetrics F20 as a function of annealing time. Once the film thickness of the nanocomposite thin film reached the desired value, the chamber was opened and the CHCl 3 vapour was allowed to freely evaporate. TEM To prepare the cross-section of a nanocomposite thin film for TEM imaging, the sample was floated off from the substrate on the surface of a pool of 5 vol% hydrogen fluoride solution. An epoxy block (Araldite 502, Electron Microscopy Sciences) was used to catch the film such that the sample is on top of the epoxy block with the air/polymer interface in contact with the epoxy block. The epoxy along with the sample were cured at 60 °C for at least 4 h to ensure good contact between the epoxy and the nanocomposite thin film. Thin sections, ∼ 50 nm in thickness, were microtomed using an RMC MT-X ultramicrotome (Boeckler Instruments) and picked up on copper TEM grids on top of water. The cross-sectional TEM images were collected using a FEI Tecnai 12 transmission electron microscope at an accelerating voltage of 120 kV. In situ GISAXS measurements GISAXS measurements were made at beamline 8-ID-E in Advanced Photon Source in Argonne National Laboratory. X-ray wavelength of 1.687 Å was used and the scattering spectra were collected on a Pilatus 1M detector (Pilatus) during solvent annealing at an incident angle larger than the critical angle of the Si substrate, usually around 0.25°. With CHCl 3 vapour in the annealing chamber, the exposure time was chosen to be shorter than 5 s to avoid serious beam damage on the film. Line averaged intensities were reported as I versus q , where q =(4 π / λ ) sin(θ/2), λ is the wavelength of incident X-rays, and θ is the scattering angle. AFM AFM was performed on a Veeco Dimension 3100 equipped with a NanoScope IIIa controller and Quadrex signal processor. The spring constant of the cantilever was 10–130 N m −1 with a resonant frequency in the range of 250–400 kHz. The set point for autotune was 2.5 V. The set-point amplitude was 90% of the free vibration value. Optical property measurements Reflection ellipsometry experiment was conducted using a spectroscopic ellipsometer (M2000U, J.A. Woollam) to measure the complex refractive index of the as-cast and annealed supramolecular nanocomposite thin films ( Supplementary Table 1 ). The white light source used had a broad spectrum of wavelength ranging from 250 to 1,000 nm. When the light source is perpendicular to the sample, the diameter of the incident light spot was around 2 mm. At incident angle 75°, the spot size increased to 6 mm in the projection direction. Biaxial model was used to retrieve the refractive index of the samples. The fitting had small mean square error (<5), which confirms the reliability of the retrieved data. Fabrication of lithographic trench pattern The rectangular trenches were fabricated using e-beam lithography and have average width and height around 135 and 50 nm, respectively. How to cite this article: Kao, J. et al . Rapid fabrication of hierarchically structured supramolecular nanocomposite thin films in 1 min. Nat. Commun. 5:4053 doi: 10.1038/ncomms5053 (2014).